Cytosolic targeting factor AKR2A captures chloroplast outer membrane-localized client proteins at the ribosome during translation In eukaryotic cells, organellar proteome biogenesis is pivotal for cellular function. Chloroplasts contain a complex proteome, the biogenesis of which includes post-translational import of nuclear-encoded proteins. However, the mechanisms determining when and how nascent chloroplast-targeted proteins are sorted in the cytosol are unknown. Here, we establish the timing and mode of interaction between ankyrin repeat-containing protein 2 (AKR2A), the cytosolic targeting factor of chloroplast outer membrane (COM) proteins, and its interacting partners during translation at the single-molecule level. The targeting signal of a nascent AKR2A client protein residing in the ribosomal exit tunnel induces AKR2A binding to ribosomal RPL23A. Subsequently, RPL23A-bound AKR2A binds to the targeting signal when it becomes exposed from ribosomes. Failure of AKR2A binding to RPL23A in planta severely disrupts protein targeting to the COM; thus, AKR2A-mediated targeting of COM proteins is coupled to their translation, which in turn is crucial for biogenesis of the entire chloroplast proteome. Chloroplast proteome biogenesis involves the import of a large number of nuclear-encoded proteins from the cytosol after translation. More than 3,000 proteins are targeted to chloroplasts from the cytosol by multiple pathways [1] , [2] , [3] . The main focus of studies on chloroplast targeting has been to elucidate the mechanisms that mediate transfer of the transit peptide-containing precursors across two envelope membranes. During passage across the membranes, the precursors bind to surface-localized receptors, such as Toc159, Toc33 and Toc34, and subsequently translocate through the import channels Toc75 and Tic20 at the outer and inner envelope membranes, respectively. At the stromal side of the inner membrane, complexes containing Tic110-Tic40-Hsp93 or cpHsp70 interact with incoming precursors to mediate the translocation activity [4] , [5] , [6] , [7] . How nascent chloroplast proteins are specifically recognized in the cytosol after translation is not completely known. Sorting is the earliest step in organellar protein targeting. Recent work identified Arabidopsis ankyrin repeat-containing protein 2 (AKR2), AKR2A and AKR2B as cytosolic targeting factors for chloroplast outer membrane (COM) proteins [8] , [9] , [10] . These COM proteins are involved in chloroplast functions including protein import and communication between the chloroplast and cytosol; therefore, AKR2A-mediated protein targeting directly or indirectly plays a crucial role in all chloroplast activities. In this study, we investigated when and how AKR2A specifically recognized its nascent cargo proteins in the cytosol during protein targeting to chloroplasts. We employed atomic force microscopy (AFM) and measured the interaction between corresponding partners at the single-molecule level. AFM force measurement and mapping have been useful for studying single-molecule recognition events [11] , [12] , [13] , [14] , [15] , [16] , [17] , [18] , [19] , [20] . We reported previously that the dendron-modified surface generated sufficient lateral spacing between immobilized biomolecules, thereby improving biomolecular detection with a greater tendency to observe force curves with single-rupture event [21] , [22] , [23] , [24] , [25] . The current study presents evidence that the targeting signal of nascent AKR2A clients residing in the ribosomal exit tunnel induces AKR2A binding to ribosomal RPL23A at an early stage of translation, whereas AKR2A binds simultaneously to RPL23A and the exposed targeting signal emerging from the exit tunnel at a later stage of translation. RPL23A artificial microRNA (amiRNA) plants, which have low RPL23A levels, have an albino phenotype with defective protein targeting to the COM, stroma and thylakoids. AKR2A binds to ribosomes that translate its client proteins The first event in AKR2A-mediated protein targeting to chloroplasts is to sort the client proteins from the pool of nascent proteins in the cytosol. To gain insight into the sorting mechanism, we examined when AKR2A binds to its clients. We hypothesized that the earliest binding occurs during translation because AKR2A recognizes the hydrophobic transmembrane domain (TMD) of client proteins, which may require AKR2A binding to ribosomes. To test this, wheat-germ extracts were incubated with His:AKR2A, and proteins bound to ribosomes were precipitated and analysed by western blotting using an anti-His antibody. His:green fluorescent protein (GFP) was included as a negative control. His:AKR2A, but not His:GFP, was detected in the precipitates, indicating that AKR2A binds to ribosomes ( Fig. 1a ). This result prompted us to examine whether AKR2A binds to its clients during translation. Ribosome-nascent chain complexes (RNCs) of chloroplast outer envelope protein 7 (OEP7), RNC-OEP7, were prepared by translating OEP7 as an AKR2A client in wheat-germ extracts. The termination codon of OEP7 was removed to prevent release from ribosomes [26] . OEP7 was labelled with [ 35 S]methionine and [ 35 S]cysteine. A 7.0 kDa protein band was detected by autoradiography, confirming OEP7 translation. Next, RNC-OEP7 was precipitated from wheat-germ extracts by ultracentrifugation, and the presence of His:AKR2A in the pellet was examined by western blot analysis using an anti-His antibody. His:AKR2A was detected in the pellet fraction ( Fig. 1a ). The amount of His:AKR2A in the pellets was higher with RNC-OEP7 than with no DNA ( Fig. 1a ), indicating that OEP7 translation enhances AKR2A binding to RNC-OEP7. In a reciprocal experiment, the incubation mixtures were subjected to immunoprecipitation (IP) with an anti-His antibody. To test for the presence of ribosomes, the immunoprecipitates were examined for the presence of 18S rRNA using RT-PCR. The 18S rRNA was detected in precipitates from mixtures that had been incubated with His:AKR2A, but not in those incubated with His:GFP ( Fig. 1b ). This result is consistent with the hypothesis that AKR2A is recruited to ribosomes for client binding during translation. In fact, the AKR2A ankyrin repeat domain (ARD) is sufficient for ribosome binding ( Supplementary Fig. 1 ). 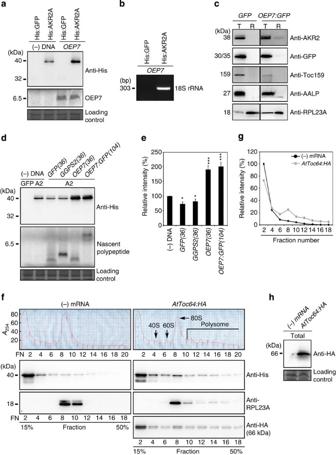Figure 1: AKR2A is recruited to ribosomes during translation. (a,b) His:AKR2A binding to ribosomes or RNC-OEP7. (a) Wheat-germ extracts were incubated withOEP7or without DNA [(−)DNA] in the presence of His:AKR2A or His:GFP. The ribosome fractions were analysed by western blotting. OEP7 was labelled with [35S]methionine and [35S]cysteine. Lower panel: loading control shows a segment of the Coomassie blue-stained blot. (b) The presence of 18S rRNA in the immunoprecipitates was detected by RT-PCR using 18S rRNA-specific primers. (c) RNC binding of endogenous AKR2s. Protoplasts were transformed withOEP7:GFPorGFP. Total extracts and RNC fractions were analysed by western blotting using the indicated antibodies. R=RNC fraction; T=total extracts. (d,e) Specific binding of AKR2A to RNCs with chloroplast outer membrane proteins. (d) Wheat-germ extracts were incubated with the indicated constructs or no DNA in the presence of His:AKR2A or His:GFP, and ribosomes or RNC fractions were analysed by western blotting. GFP, His:GFP; A2, His:AKR2A; Loading control, a segment of the Coomassie blue-stained blot. (e) To quantify His:AKR2A binding to RNCs, the His:AKR2A band signal intensity was measured using LAS3000 and software (FUJIFILM). The signal intensity of His:AKR2A is a value (%) relative to that of (-) DNA. Mean±s.d. are shown (n=3). Asterisks indicate a significant difference from the corresponding control experiment by Student’st-test (*P<0.05; **P<0.01; ***P<0.001). (f–h) AKR2A association with translating ribosomes. (f) His:AKR2A together withAtToc64:HAmRNA or no mRNA were added to the wheat-germ extracts. After ultracentrifugation on a linear sucrose gradient, the fractions were analysed by western blotting using anti-His, anti-HA and anti-RPL23A antibodies. (-) mRNA=no mRNA; FN=fraction number; 40S=40S ribosomes; 60S=60S ribosomes; and 80S=80S ribosomes. (g) To quantify the amount of His:AKR2A in these fractions, the signal intensity of His:AKR2A bands was measured and presented as a relative value (%) to that in fraction 2 of (-) mRNA. (h) To confirm translation of AtToc64:HA, 5% of the translation mixture in (f) was analysed by western blotting using an anti-HA antibody. Loading control, a protein band of the immunoblot stained with Coomassie blue. Figure 1: AKR2A is recruited to ribosomes during translation. ( a , b ) His:AKR2A binding to ribosomes or RNC-OEP7. ( a ) Wheat-germ extracts were incubated with OEP7 or without DNA [(−)DNA] in the presence of His:AKR2A or His:GFP. The ribosome fractions were analysed by western blotting. OEP7 was labelled with [ 35 S]methionine and [ 35 S]cysteine. Lower panel: loading control shows a segment of the Coomassie blue-stained blot. ( b ) The presence of 18S rRNA in the immunoprecipitates was detected by RT-PCR using 18S rRNA-specific primers. ( c ) RNC binding of endogenous AKR2s. Protoplasts were transformed with OEP7:GFP or GFP . Total extracts and RNC fractions were analysed by western blotting using the indicated antibodies. R=RNC fraction; T=total extracts. ( d , e ) Specific binding of AKR2A to RNCs with chloroplast outer membrane proteins. ( d ) Wheat-germ extracts were incubated with the indicated constructs or no DNA in the presence of His:AKR2A or His:GFP, and ribosomes or RNC fractions were analysed by western blotting. GFP, His:GFP; A2, His:AKR2A; Loading control, a segment of the Coomassie blue-stained blot. ( e ) To quantify His:AKR2A binding to RNCs, the His:AKR2A band signal intensity was measured using LAS3000 and software (FUJIFILM). The signal intensity of His:AKR2A is a value (%) relative to that of (-) DNA. Mean±s.d. are shown ( n =3). Asterisks indicate a significant difference from the corresponding control experiment by Student’s t -test (* P <0.05; ** P <0.01; *** P <0.001). ( f – h ) AKR2A association with translating ribosomes. ( f ) His:AKR2A together with AtToc64:HA mRNA or no mRNA were added to the wheat-germ extracts. After ultracentrifugation on a linear sucrose gradient, the fractions were analysed by western blotting using anti-His, anti-HA and anti-RPL23A antibodies. (-) mRNA=no mRNA; FN=fraction number; 40S=40S ribosomes; 60S=60S ribosomes; and 80S=80S ribosomes. ( g ) To quantify the amount of His:AKR2A in these fractions, the signal intensity of His:AKR2A bands was measured and presented as a relative value (%) to that in fraction 2 of (-) mRNA. ( h ) To confirm translation of AtToc64:HA, 5% of the translation mixture in ( f ) was analysed by western blotting using an anti-HA antibody. Loading control, a protein band of the immunoblot stained with Coomassie blue. Full size image We tested the binding of endogenous AKR2s to RNCs. Protoplasts were transformed with OEP7:GFP targeted to COM, or GFP as a control, and RNCs were pelleted from protoplast extracts by ultracentrifugation. Endogenous AKR2s were detected in the pellet from extracts of protoplasts expressing OEP7:GFP but not transformed with GFP ( Fig. 1c ), thereby confirming that AKR2s bind to RNCs with OEP7:GFP. Ribosomal enrichment in the pellet fraction with little contamination from chloroplasts and soluble proteins was confirmed by western blot analyses using anti-RPL23A, anti-Toc159 and anti-AALP antibodies, respectively. To determine when AKR2A binds to RNCs containing AKR2A clients, RNCs were prepared with two different polypeptide lengths; OEP7(36) and OEP7:GFP(104) had 36 and 104 amino-acid (aa) residues, including the two targeting signal components, TMD, and C-terminal positively charged flanking region (CPR). The entire OEP7(36) nascent chain should be located within the ribosomal exit tunnel, whereas the N-terminal OEP7 moiety of the OEP7:GFP(104) nascent chain should be exposed from the ribosomal exit tunnel. Both OEP7(36) and OEP7:GFP(104) without the termination codon were translated using the wheat-germ extracts in the presence of His:AKR2A. RNCs were precipitated by ultracentrifugation and analysed by western blotting using an anti-His antibody ( Fig. 1d,e ). For controls, wheat-germ extracts were incubated with no DNA in the presence of His:AKR2A or GFP. The amount of His:AKR2A coprecipitated with RNC-OEP7:GFP(104) was two-fold higher than that of the vacant ribosomes. The level of His:AKR2A binding to RNC-OEP7(36) increased to approximately the same level as that binding to RNC-OEP7:GFP(104). To confirm the strong binding of His:AKR2A to RNC-OEP7(36), we tested His:AKR2A binding with another COM protein AtToc64 [27] and with non-chloroplast proteins. His:AKR2A showed strong binding to RNC-AtToc64(36). By contrast, His:AKR2A exhibited slightly reduced binding (relative to binding to the vacant ribosomes) to RNCs containing 36 aa non-chloroplast proteins, including cytosolic GFP(36), geranylgeranyl pyrophosphate synthase 2(36) [GGPS2(36); endoplasmic reticulum (ER) membrane protein] and binding protein (36) [BiP(36); ER lumenal protein] ( Fig. 1d,e and Supplementary Fig. 2 ). These results confirm that AKR2A specifically binds to RNCs containing chloroplast outer membrane proteins. Translation of all six constructs was confirmed by autoradiography ( Fig. 1d and Supplementary Fig. 2 ). To further test the association of AKR2A with translating ribosomes, we fractionated the in vitro translation mixtures on a sucrose gradient and examined the distribution profile of His:AKR2A and ribosomes on the gradient. Here, we used the 64 kDa HA-tagged AtToc64 ( AtToc64:HA ) as the AKR2A client because OEP7 is too short to produce polysomes. Wheat-germ extracts were incubated with AtToc64:HA mRNA or without mRNA in the presence of His:AKR2A, and fractionated on a 15−50% linear sucrose gradient by ultracentrifugation. The gradient fractions were analysed for ribosomes by measuring absorbance at 254 nm ( A 254 ) ( Fig. 1f ); these results were confirmed by western blot analysis using an anti-RPL23A antibody. Without mRNA, the majority of RPL23A was detected in fraction numbers 8 and 10, which contained monosomes; this result was consistent with the A 254 profile. With AtToc64:HA mRNA, the majority of RPL23A was detected in the monosome fractions but at substantially lower levels than that of the translation mixture without mRNA; concomitantly, the RPL23A intensity was higher in the polysome fractions. Next, we detected His:AKR2A in these fractions. Without mRNA, His:AKR2A was found primarily in the top fraction, with little or no His:AKR2A visible in the monosome or polysome fractions. With AtToc64:HA mRNA, the amount of His:AKR2A in the top fraction decreased, and the amount in monosome and polysome fractions concomitantly increased ( Fig. 1f,g ). The distribution of His:AKR2A closely coincided with that of AtToc64:HA ( Fig. 1f ). These results confirm that AKR2A associates with translating ribosomes. Translation of AtToc64:HA was confirmed by western blot analysis using an anti-HA antibody ( Fig. 1h ). Collectively, these results strongly support the hypothesis that AKR2A captures its clients at ribosomes during translation. AKR2A specifically recognizes its clients on the ribosome We tested the interaction between AKR2A and RNC-OEP7(36) at the single-molecule level using AFM. RNC-GGPS2(36) and RNC-GFP(36) were included as negative controls. To confirm translation of these constructs, the translation mixtures were subjected to sodium dodecyl sulfate–PAGE (SDS–PAGE) and protein bands were detected by autoradiography ( Fig. 2a ). For AFM experiments, the third-generation dendron was introduced onto the probe and the substrate through a self-assembly process to generate appropriate spacing between proteins on the surface of the probe and between RNCs on the substrate surface. Appropriate linkers were employed to provide controlled orientation of both substrate and probe. For AFM experiments, RNCs were immobilized on the streptavidin-modified substrate using biotinyl groups incorporated into mRNA. Conversely, AKR2A was immobilized on the reduced glutathione (GSH)-tethered AFM tip by fusing the AKR2A N-terminus to glutathione S -transferase (GST); this fusion site is distant from the AKR2A ribosome-binding domain ( Fig. 2b ). Therefore, immobilization of AKR2A and translating ribosomes to the AFM tip and substrate, respectively, should not interfere with the interaction between AKR2A and ribosomes during the AFM force measurements. 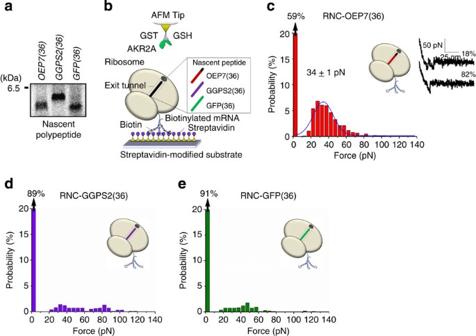Figure 2: Nascent AKR2A client chain induces AKR2A binding to RNCs before emergence from the exit tunnel. (a) Translation of the indicated cargoes in wheat-germ extracts. RNCs were precipitated by ultracentrifugation and separated by SDS–PAGE followed by autoradiography. Nascent polypeptides were labelled with [35S]methionine and [35S]cysteine. (b) Schematic of the experimental set-up. GST-fused AKR2A was immobilized onto the AFM tip, and RNCs containing biotinylated mRNA were immobilized onto the dendron-modified surface. RNCs were prepared from wheat-germ extracts by translating OEP7(36), GGPS2(36) or GFP(36) without the termination codon. (c–e) Force histograms of the specific interaction between AKR2A and RNCs. Histograms were obtained from the whole set of specific curves for RNC-OEP7(36) (n=1,040) (c), RNC-GGPS2(36) (n=1,011) (d) and RNC-GFP(36) (n=1,082) (e). The value indicated by an arrow is the probability of no unbinding event. Gaussian fitting gave the most probable unbinding force and representative force-distance curves were shown for RNC-OEP7(36). Figure 2: Nascent AKR2A client chain induces AKR2A binding to RNCs before emergence from the exit tunnel. ( a ) Translation of the indicated cargoes in wheat-germ extracts. RNCs were precipitated by ultracentrifugation and separated by SDS–PAGE followed by autoradiography. Nascent polypeptides were labelled with [ 35 S ]methionine and [ 35 S ]cysteine. ( b ) Schematic of the experimental set-up. GST-fused AKR2A was immobilized onto the AFM tip, and RNCs containing biotinylated mRNA were immobilized onto the dendron-modified surface. RNCs were prepared from wheat-germ extracts by translating OEP7(36), GGPS2(36) or GFP(36) without the termination codon. ( c – e ) Force histograms of the specific interaction between AKR2A and RNCs. Histograms were obtained from the whole set of specific curves for RNC-OEP7(36) ( n =1,040) ( c ), RNC-GGPS2(36) ( n =1,011) ( d ) and RNC-GFP(36) ( n =1,082) ( e ). The value indicated by an arrow is the probability of no unbinding event. Gaussian fitting gave the most probable unbinding force and representative force-distance curves were shown for RNC-OEP7(36). Full size image Unbinding force histograms were analysed by fitting with a single Gaussian curve, in which the most probable force value was 34±1 pN (mean±s.e.m. ; n =1,040) for RNC-OEP7(36) ( Fig. 2c ). By contrast, the force histograms of RNC-GGPS2(36) ( n =1,011) and RNC-GFP(36) ( n =1,081) ( Fig. 2d,e ) did not fit with the single Gaussian curve, which indicated that the unbinding event probability was lower than that of RNC-OEP7(36). The significance of the average force value differences between RNC-OEP7(36) and RNC-GGPS2(36) and between RNC-OEP7(36) and RNC-GFP(36) was examined by t -test. The difference was considered to be statistically significant ( P <0.01) for RNC-OEP7(36) but not for RNC-GGPS2(36) or RNC-GFP(36). This indicates that AKR2A binds to RNC-OEP7(36) but not to RNC-GGPS2(36) or RNC-GFP(36). As a control for the RNCs containing biotinylated mRNA, wheat-germ extracts were incubated without mRNA before applying to the substrate, and then subjected to AFM. AKR2A did not interact with this control, confirming that vacant ribosomes do not bind to the streptavidin-modified substrate ( Supplementary Fig. 3 ). These results suggest that AKR2A differentiates its binding ribosomes depending on the type of nascent chains undergoing translation, even when they are located in the ribosomal exit tunnel. AKR2A simultaneously binds to ribosomes and nascent chain We examined AKR2A binding to RNCs when its clients were exposed from ribosomes. A previous study showed that the AKR2A N-terminal domain binds to OEP7 [8] . As a reference, the unbinding force-distance curves between AKR2A and OEP7 were recorded using AFM. The OEP7 targeting signal contains two components, TMD (aa positions 10−27) and CPR (aa positions 28−36). We generated four serial deletion mutants designated OEP7(9), OEP7(27), OEP7(36) and OEP7(50). OEP7(9) did not contain the targeting signal, OEP7(27) contained only TMD but lacked CPR, and OEP7(36) and OEP7(50) contained both TMD and CPR. GST-fused OEP7 deletion constructs and GST:AKR2A were immobilized onto the GSH-modified substrate and GSH-tethered tip, respectively ( Supplementary Fig. 4a–e ). Unbinding force histograms were analysed by fitting with the single Gaussian curve. The most probable force values were 40±1 pN (mean±s.e.m. ; n =1,090), 40±1 pN (mean±s.e.m. ; n =1,030) and 32±1 pN (mean±s.e.m. ; n =1,008) for the interactions with AKR2A-OEP7(50), AKR2A-OEP7(36) and AKR2A-OEP7(27), respectively ( Supplementary Fig. 4f–h ). AKR2A-OEP7(27) had a slightly lower interaction force than that of the other two interactions, which may be due to the absence of CPR in OEP7(27). By contrast, the unbinding force value of OEP7(9) was lower than those of the other three deletion mutants and the histogram did not fit the single Gaussian curve; the specific unbinding event probability was reduced to 18% ( Supplementary Fig. 4i ). These results confirm that both TMD and CPR in the targeting signal contribute to AKR2A binding OEP7. Next, we examined the mode of AKR2A interaction with RNC-OEP7:GFP(90), in which the targeting signal of OEP7:GFP(90) was exposed from ribosomes, and compared it with that of RNC-OEP7(36), in which the entire nascent chain of OEP7(36) resided within the ribosomal exit tunnel. AKR2A and RNCs were immobilized onto the tip and substrate, respectively ( Fig. 3a ). The most probable force value and stretching-distance value for RNC-OEP7(36) were 34±1 pN and 4±1 nm (mean±s.e.m. ; n =1,040), respectively ( Fig. 2c and Supplementary Fig. 5a ), whereas for RNC-OEP7:GFP(90) they were 42±1 pN and 10±1 nm (mean±s.e.m. ; n =1,121), respectively ( Fig. 3b and Supplementary Fig. 5b ). The unbinding force curves show a double peak with 18 and 38% probability for RNC-OEP7(36) and RNC-OEP7:GFP(90), respectively ( Figs 2c and 3b and Supplementary Fig. 6 ). The double peak in the unbinding curves represents two independent interactions between the two binding partners, raising the possibility that AKR2A has two interactions with RNCs. However, a difference in the probability of the double-peaked events between the two samples suggests that the nature of the two interactions between AKR2A and RNCs may not be identical. AKR2A has two binding domains, the N-terminal domain for binding the targeting signal [8] and the ARD for binding the ribosome ( Supplementary Fig. 1 ). RNC-OEP7:GFP(90) may also have two binding sites (the OEP7 targeting signal and the ribosome) for AKR2A; thus, for RNC-OEP7:GFP(90), one interaction may occur between the N-terminal domain of AKR2A and OEP7:GFP(90) [8] , and the other interaction may occur between the ARD and ribosomes. By contrast, for RNC-OEP7(36), both interactions should occur between AKR2A and ribosomes. 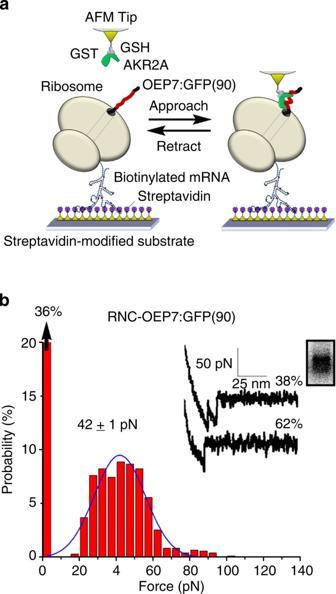Figure 3: Unbinding force-distance curves show that AKR2A simultaneously binds to ribosome and nascent chain of RNC-OEP7:GFP(90) during translation. (a) Schematic for measuring the interaction between AKR2A and RNC-OEP7:GFP(90). (b) Force histograms and representative force-distance curves. Histograms were obtained from the whole set of specific curves for the interaction between AKR2A and RNC-OEP7:GFP(90) (n=1,121). The value indicated by an arrow is the probability of no unbinding events. Gaussian fitting gave the most probable unbinding force. Inset confirmsOEP7:GFP(90)translation by SDS–PAGE and autoradiography. Figure 3: Unbinding force-distance curves show that AKR2A simultaneously binds to ribosome and nascent chain of RNC-OEP7:GFP(90) during translation. ( a ) Schematic for measuring the interaction between AKR2A and RNC-OEP7:GFP(90). ( b ) Force histograms and representative force-distance curves. Histograms were obtained from the whole set of specific curves for the interaction between AKR2A and RNC-OEP7:GFP(90) ( n =1,121). The value indicated by an arrow is the probability of no unbinding events. Gaussian fitting gave the most probable unbinding force. Inset confirms OEP7:GFP(90) translation by SDS–PAGE and autoradiography. Full size image To gain insight into the interaction that produces the double peak in the unbinding event, we examined the binding of AKR2A to RNCs using AFM mapping. Force mapping measures key parameters including cluster size, stretching distance, unbinding force value and unbinding probability, and these parameters can be used to confirm the interaction type [28] , [29] , [30] , [31] . Adhesion force maps were obtained for a 300 nm × 300 nm area, and the unbinding force was recorded at 15-min intervals with five measurements at each pixel. The pixel size was chosen as smaller than the expected hydrodynamic distance of RNCs attached to the substrate. In this way, individual RNCs would appear as a cluster in the force map. The dimension of 80S ribosomes is 30 nm × 31 nm × 20 nm (height × width × thickness) [32] , and biotinylated mRNA should also contribute to the hydrodynamic distance; therefore, the chosen pixel size (15 nm) should be smaller than the hydrodynamic diameter. In the force maps, pixels showing the specific unbinding curve more than twice were included ( Supplementary Fig. 7 ), whereas pixels showing the specific unbinding curve only once were discarded (black in the map). The force level of each pixel in the map was determined by the average unbinding force value. Specific pixels were categorized into three groups: light grey (≤ 13 pN), yellow (14−70 pN) and orange (≥ 71 pN). Because the most probable force value for the interaction between AKR2A and RNC-OEP7:GFP(90) was 42 pN, and the s.d. was 14 pN, the yellow group ranged from 14 (42–2 × 14) pN to 70 (42+2 × 14) pN. A cluster containing more than five yellow pixels connected to each other within a boundary was selected to assign the RNCs in the map. Four clusters of RNC-OEP7(36) and three clusters of RNC-OEP7:GFP(90) were evident in representative force maps ( Fig. 4a,b ). Within these clusters, double-peaked unbinding events that were recorded more than once were indicated by an asterisk. The percentage of pixels marked with an asterisk was significantly larger with RNC-OEP7:GFP(90) (C1, 62%; C2, 57%; and C3, 78%) than with RNC-OEP7(36) (C1, 14%; C2, 33%; C3, 0%; and C4, 18%) ( Fig. 4c,d ). 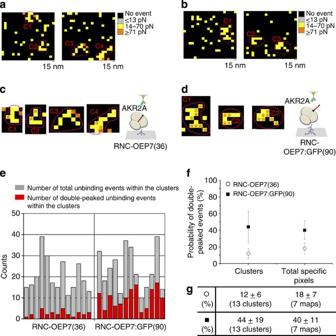Figure 4: Adhesion force analysis and mapping indicate two sites of AKR2A binding to RNCs when nascent AKR2A client chain emerges from the ribosomal exit tunnel. (a,b) Adhesion force maps for the interaction between AKR2A and RNCs. Force maps were obtained for RNC-OEP7(36) (a) and RNC-OEP7:GFP(90) (b) after the filtering process. The unbinding force value of each pixel was colour-coded according to the scale shown in the inset on the right. (c,d) Zoomed-in maps of RNC-OEP7(36) (c) and RNC-OEP7:GFP(90) (d). Asterisks indicate double-peaked unbinding events detected within the corresponding cluster. Inset on the right, schematic drawing of the interaction. (e) Number of total unbinding events within a cluster (grey) and number of double-peaked unbinding events (red). A total of 13 clusters for each case were compared. (f,g) Probability of the double-peaked events for RNC-OEP7(36) and RNC-OEP7:GFP(90). (f) Probability for the double-peaked event within both clusters and the total specific pixels. (g) Comparison of the averaged probability of the double-peaked events for RNC-OEP7(36) and RNC-OEP7:GFP(90). Figure 4: Adhesion force analysis and mapping indicate two sites of AKR2A binding to RNCs when nascent AKR2A client chain emerges from the ribosomal exit tunnel. ( a , b ) Adhesion force maps for the interaction between AKR2A and RNCs. Force maps were obtained for RNC-OEP7(36) ( a ) and RNC-OEP7:GFP(90) ( b ) after the filtering process. The unbinding force value of each pixel was colour-coded according to the scale shown in the inset on the right. ( c , d ) Zoomed-in maps of RNC-OEP7(36) ( c ) and RNC-OEP7:GFP(90) ( d ). Asterisks indicate double-peaked unbinding events detected within the corresponding cluster. Inset on the right, schematic drawing of the interaction. ( e ) Number of total unbinding events within a cluster (grey) and number of double-peaked unbinding events (red). A total of 13 clusters for each case were compared. ( f , g ) Probability of the double-peaked events for RNC-OEP7(36) and RNC-OEP7:GFP(90). ( f ) Probability for the double-peaked event within both clusters and the total specific pixels. ( g ) Comparison of the averaged probability of the double-peaked events for RNC-OEP7(36) and RNC-OEP7:GFP(90). Full size image To further examine the probability of the double-peaked unbinding events, seven maps for each sample were obtained, and thirteen clusters for each RNC were analysed in detail ( Supplementary Tables 1 and 2 ). For three representative clusters of RNC-OEP7(36) (C1, C10 and C13), the measured values of the stretching distance, unbinding force and unbinding probability were converted to the corresponding contour maps ( Supplementary Fig. 8 ). Although the overall behaviour matched with that in a previous study for DNAs [31] , the shape of the clusters was far from ellipsoid and the clusters were multi-centred, indicating complexity in the hydrodynamic movement of the surface-bound RNCs. For each cluster, the total number of specific events within the clusters and the number of double-peaked unbinding events in the pixels with asterisks were displayed for comparison ( Fig. 4e ). The probability of pixels with an asterisk was much higher with RNC-OEP7:GFP(90) than with RNC-OEP7(36). To confirm this, we compared the probability of the double-peaked curves with respect to the total specific curves within the clusters. The probability was 44±19% and 12±6% for RNC-OEP7:GFP(90) and RNC-OEP7(36), respectively ( Fig. 4f,g , left). When the noncluster-forming pixels were included in the calculation, the probability of the double-peaked events was 40±11% and 18±7% for RNC-OEP7:GFP(90) and RNC-OEP7(36), respectively ( Fig. 4f,g , right). These results show that RNC-OEP7:GFP(90) had a much higher probability than RNC-OEP7(36) to produce double-peaked curves in the unbinding events. By contrast, the probability of specific events was similar for both samples: 53±8% for RNC-OEP7:GFP(90) and 53±10% for RNC-OEP7(36) ( Supplementary Table 3 ). One possible explanation for these results is that both of the two interactions between AKR2A and RNC-OEP7:GFP(90) are specific, whereas only one of the two interactions between AKR2A and RNC-OEP7(36) is specific. AKR2A binds to ribosomal RPL23A We defined the ribosomal binding site for AKR2A. RPL23 is located near the exit site of the ribosomal tunnel and interacts with various factors such as SRP, nascent-chain associated complex (NAC) and Trigger factor [33] , [34] , [35] , [36] , [37] . Therefore, RPL23 appears to serve as a general docking site for cytosolic factors that transiently associate with ribosomes to mediate protein targeting or folding of nascent polypeptide. RPL23 is one of the strong candidates for the ribosomal docking site for AKR2A binding. We examined AKR2A binding to two isoforms of RPL23A, RPL23aA and RPL23aB, which are Arabidopsis orthologues of RPL23 [38] . GST:AKR2A was incubated with His:RPL23aA or His:RPL23aB, and proteins were precipitated and analysed by western blotting using an anti-His antibody ( Fig. 5a ). AKR2A bound to both RPL23aA and RPL23aB, but with stronger affinity to RPL23aB. The interaction between AKR2A and RPL23aA or RPL23aB was examined at the single-molecule level by AFM. The most probable force values were 32±1 pN (mean±s.e.m. ; n =1,130) and 30±1 pN (mean±s.e.m. ; n =1,032), respectively ( Supplementary Fig. 9 ). The observed probability of an unbinding event for RPL23aB was higher than that for RPL23aA. In addition, to understand the dissociation energy landscape and the kinetics, the loading dependence of the two reference systems [AKR2A-RPL23aB and AKR2A-OEP7(36)] was studied, which revealed that single-energy barriers existed for both interactions; the kinetic off-rate constant ( k off ) and the energy barrier distance ( x β ) were 2.01±1.22 s −1 and 0.92±0.30 nm for the AKR2A-RPL23aB interaction and 0.53±0.14 s −1 and 0.86±0.14 nm for the AKR2A-OEP7(36) interaction, respectively ( Supplementary Fig. 10 and Supplementary Table 4 ). The values are within the published ranges of off-rate constants and length scales of other proteins [22] , [39] , [40] , [41] . 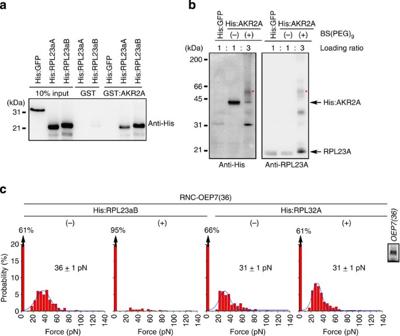Figure 5: AKR2A binds to RPL23A located at the ribosomal exit site during translation. (a)In vitropull-down experiments of AKR2A with RPL23aA and RPL23aB. GST:AKR2A, His:RPL23aA and His:RPL23aB constructs were expressed inE. coliand purified using affinity chromatography. GST:AKR2A (3 μg) immobilized on glutathione-agarose beads was incubated with His:RPL23aA or His:RPL23aB (1 μg) at 4 °C for 3 h, and proteins were precipitated with glutathione-agarose beads. GST alone and His:GFP were included as controls. The precipitates were analysed by western blotting using an anti-His antibody. (b) Crosslinking of AKR2A to RPL23A on ribosomes. TheOEP7(36)construct was translated in the wheat-germ translation system in the presence of His:AKR2A and treated with BS(PEG)9. RNC-OEP7(36) was separated by ultracentrifugation and analysed by western blotting using an anti-His antibody. The immunoblot was stripped and redetected with an anti-RPL23A antibody. Asterisk designates the band recognized by both anti-His and anti-RPL23A antibodies. Loading ratio, the ratio of the loading amounts of proteins in each lane. (c) Specificity of the interaction between AKR2A and RPL23A. Force histograms of the interaction between AKR2A and RNC-OEP7(36) were obtained in the presence (+) and absence (−) of 0.5 μM His:RPL23aB (n=688 and 648, respectively) or 0.5 μM His:RPL32A (n=697 and 646, respectively, used as a negative control). The value indicated by an arrow is the probability of no unbinding events. Gaussian fitting gave the most probable unbinding force. Inset, translation ofOEP7(36)confirmed by SDS–PAGE and autoradiography. Figure 5: AKR2A binds to RPL23A located at the ribosomal exit site during translation. ( a ) In vitro pull-down experiments of AKR2A with RPL23aA and RPL23aB. GST:AKR2A, His:RPL23aA and His:RPL23aB constructs were expressed in E. coli and purified using affinity chromatography. GST:AKR2A (3 μg) immobilized on glutathione-agarose beads was incubated with His:RPL23aA or His:RPL23aB (1 μg) at 4 °C for 3 h, and proteins were precipitated with glutathione-agarose beads. GST alone and His:GFP were included as controls. The precipitates were analysed by western blotting using an anti-His antibody. ( b ) Crosslinking of AKR2A to RPL23A on ribosomes. The OEP7(36) construct was translated in the wheat-germ translation system in the presence of His:AKR2A and treated with BS(PEG) 9 . RNC-OEP7(36) was separated by ultracentrifugation and analysed by western blotting using an anti-His antibody. The immunoblot was stripped and redetected with an anti-RPL23A antibody. Asterisk designates the band recognized by both anti-His and anti-RPL23A antibodies. Loading ratio, the ratio of the loading amounts of proteins in each lane. ( c ) Specificity of the interaction between AKR2A and RPL23A. Force histograms of the interaction between AKR2A and RNC-OEP7(36) were obtained in the presence (+) and absence (−) of 0.5 μM His:RPL23aB ( n =688 and 648, respectively) or 0.5 μM His:RPL32A ( n =697 and 646, respectively, used as a negative control). The value indicated by an arrow is the probability of no unbinding events. Gaussian fitting gave the most probable unbinding force. Inset, translation of OEP7(36) confirmed by SDS–PAGE and autoradiography. Full size image We performed chemical crosslinking experiments to examine whether AKR2A binds to RPL23A assembled into ribosomes. His:AKR2A was incubated with RNC-OEP7(36), and then treated with the chemical crosslinker BS(PEG) 9 . Proteins were analysed by western blotting using anti-His and anti-RPL23A antibodies ( Fig. 5b ). Without BS(PEG) 9 treatment, AKR2A and RPL23A were detected at the 40 and 20 kDa positions, respectively. After BS(PEG) 9 treatment, the amount of AKR2A was decreased from the 40 kDa position and instead was detected near the 60 kDa position. This AKR2A-positive 60 kDa band also reacted with an anti-RPL23A antibody, indicating that AKR2A binds to RPL23A assembled into the ribosome. To test the specificity of the interaction, we examined AKR2A binding to RNC-OEP7(36) in the presence of 0.5 μM His:RPL23aB as a competitor. A previous study showed that purified RPL23 specifically interacts with Trigger factor in vitro [34] . The probability of the unbinding event was reduced from 39 to 5% ( Fig. 5c , left). By contrast, when 0.5 μM His:RPL32A was used as a negative control, the probability of the unbinding event did not decrease ( Fig. 5c , right), confirming that AKR2A specifically binds to RPL23A on the ribosome. The observed most probable force values (36±1 pN (mean±s.e.m. ; n =688) and 31±1 pN (mean±s.e.m. ; n =697 or n =646)) were approximately equal to that of the interaction between AKR2A and RPL23aB. Targeting of COM proteins is impaired in knockdown plants The physiological significance of AKR2A binding to RPL23A was examined in planta . The rpl23aB mutant plants did not show any noticeable phenotype, but knockdown of both RPL23aA and RPL23aB isoforms results in a lethal phenotype [42] , [43] . To suppress both isoforms, we generated inducible RPL23A -amiRNA transgenic plants by placing RPL23A -amiRNA under the control of a dexamethasone (Dex)-inducible promoter ( Supplementary Fig. 11a ). The transcript levels of both RPL23A isoforms were significantly reduced in RPL23A -amiRNA plants when treated with 2 μM Dex ( Supplementary Fig. 11b ). Dex-treated RPL23A -amiRNA plants displayed albino or yellow-leaf phenotypes with growth defects ( Fig. 6a ) and abnormal chloroplasts lacking thylakoids and grana stacks ( Fig. 6b–g ). In addition, cells in Dex-treated RPL23A -amiRNA plants appeared to be smaller overall than those in Dex-untreated RPL23A -amiRNA plants. However, other organelles, such as mitochondria and peroxisomes, did not show any obvious visible morphological alterations at the ultrastructural level in Dex-treated RPL23A -amiRNA plants. These results indicate that RPL23A is pivotal for chloroplast biogenesis. 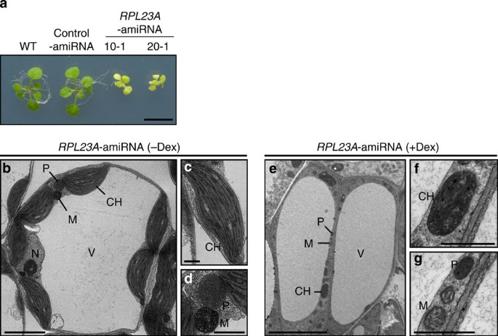Figure 6:RPL23A-amiRNA plants have defective chloroplast biogenesis. (a) Phenotype ofRPL23A-amiRNA plants. Plants were grown on Murashige-Skoog (MS) plates containing 2 μM dexamethasone for 2 weeks. Two independentRPL23A-amiRNA plant lines were analysed. WT=wild type; control-amiRNA, transgenic plants transformed with the control vector. Scale bar, 1 cm. (b–g) Chloroplast morphology inRPL23A-amiRNA plants. Ultrathin sections prepared from leaf tissues of 2-week-oldRPL23A-amiRNA plants grown in the presence and absence of 2 μM dexamethasone were examined by electron microscopy. Scale bars represent 5 μm (b,e) and 1 μm (c,d,f,g). CH=chloroplast; Dex=dexamethasone; M=mitochondrion; N=nucleus; P=peroxisome; V=vacuole. Figure 6: RPL23A -amiRNA plants have defective chloroplast biogenesis. ( a ) Phenotype of RPL23A -amiRNA plants. Plants were grown on Murashige-Skoog (MS) plates containing 2 μM dexamethasone for 2 weeks. Two independent RPL23A -amiRNA plant lines were analysed. WT=wild type; control-amiRNA, transgenic plants transformed with the control vector. Scale bar, 1 cm. ( b – g ) Chloroplast morphology in RPL23A -amiRNA plants. Ultrathin sections prepared from leaf tissues of 2-week-old RPL23A -amiRNA plants grown in the presence and absence of 2 μM dexamethasone were examined by electron microscopy. Scale bars represent 5 μm ( b , e ) and 1 μm ( c , d , f , g ). CH=chloroplast; Dex=dexamethasone; M=mitochondrion; N=nucleus; P=peroxisome; V=vacuole. Full size image We examined AKR2A binding to ribosomes in Dex-treated RPL23A -amiRNA plants. Cell extracts from control and RPL23A -amiRNA plants that had been treated with or without Dex were incubated with His:AKR2A. Ribosomes were pelleted and analysed by immunoblotting using an anti-His antibody. The amount of His:AKR2A was significantly lower in samples of Dex-treated RPL23A -amiRNA plants than in samples of Dex-treated control or Dex-untreated RPL23A -amiRNA plants ( Fig. 7a ). The levels of COM proteins Toc34, Toc75 and Toc159, a stromal protein RbcS and a thylakoid protein Lhcb4 were all lower in Dex-treated RPL23A -amiRNA plants than in the Dex-treated control or Dex-untreated RPL23A -amiRNA plants ( Fig. 7b,c ). The levels of the signal recognition particle (SRP) clients BiP, VSR and PIP2, cytosolic proteins Hsp70 and actin, and mitochondrial protein VDAC1 were not affected ( Fig. 7b,c ). The peroxisomal catalase level was reduced, although the reason for this was not clearly understood. These results strongly suggest that RPL23A plays a pivotal role in COM protein biogenesis, which, in turn, is crucial for stromal and thylakoid protein biogenesis. 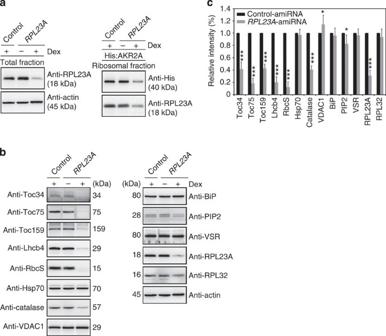Figure 7:RPL23A-amiRNA plants have a defect in COM protein targeting and chloroplast proteome biogenesis. (a) Reduced binding of His:AKR2A to ribosomes inRPL23A-amiRNA plants. Cell extracts from plants grown in the presence and absence of 2 μM dexamethasone were incubated with His:AKR2A, and ribosomes were pelleted by ultracentrifugation. Total extracts and ribosomal fractions were analysed by western blotting using an anti-His antibody. Control=control-amiRNA plants;RPL23A=RPL23A-amiRNA plants. (b,c) Effect ofRPL23Asuppression on chloroplast protein levels. (b) Protein extracts from control- andRPL23A-amiRNA plants grown under the indicated conditions were analysed by western blotting using the indicated antibodies. Loading control, actin. Control=control-amiRNA plants;RPL23A=RPL23A-amiRNA plants. (c) To quantify protein levels, the band intensity was measured using LAS3000 and software. Protein levels were normalized using actin; expression levels in control-amiRNA plants were set to 1. Mean±s.d. are shown (n=3). Asterisks indicate a significant difference from the corresponding control experiment by Student’st-test (*P<0.05; **P<0.01; ***P<0.001). Figure 7: RPL23A -amiRNA plants have a defect in COM protein targeting and chloroplast proteome biogenesis. ( a ) Reduced binding of His:AKR2A to ribosomes in RPL23A -amiRNA plants. Cell extracts from plants grown in the presence and absence of 2 μM dexamethasone were incubated with His:AKR2A, and ribosomes were pelleted by ultracentrifugation. Total extracts and ribosomal fractions were analysed by western blotting using an anti-His antibody. Control=control-amiRNA plants; RPL23A = RPL23A -amiRNA plants. ( b , c ) Effect of RPL23A suppression on chloroplast protein levels. ( b ) Protein extracts from control- and RPL23A -amiRNA plants grown under the indicated conditions were analysed by western blotting using the indicated antibodies. Loading control, actin. Control=control-amiRNA plants; RPL23A = RPL23A -amiRNA plants. ( c ) To quantify protein levels, the band intensity was measured using LAS3000 and software. Protein levels were normalized using actin; expression levels in control-amiRNA plants were set to 1. Mean±s.d. are shown ( n =3). Asterisks indicate a significant difference from the corresponding control experiment by Student’s t -test (* P <0.05; ** P <0.01; *** P <0.001). Full size image The levels of ER and plasma membrane proteins were not significantly affected in Dex-treated RPL23A -amiRNA plants. To corroborate this, we examined the extent of ribosome association with ER membranes and SRP binding to ribosomes. Cell extracts from control and Dex-treated or -untreated RPL23A -amiRNA plants were separated into soluble and microsomal fractions by ultracentrifugation, and these fractions were probed with various antibodies ( Supplementary Fig. 12 ). In Dex-treated RPL23A -amiRNA plants, the RPL23A levels in soluble and microsomal fractions were reduced. However, the SRP54 levels in microsomal fractions were the same in both Dex-treated RPL23A - and control-amiRNA plants, indicating that reduced RPL23A levels may not affect ribosomal binding of SRP. RPL29, another SRP54-binding protein at the ribosomal exit site [33] , [35] , [36] , [44] , may support SRP-mediated targeting of ER proteins in Dex-treated RPL23A -amiRNA plants ( Supplementary Fig. 12 ). In Dex-treated RPL23A -amiRNA plants, the RPL32 levels (another ribosomal protein) were not significantly different from that in control-amiRNA plants, confirming that ribosome biogenesis occurs normally. In this study, we provide compelling evidence that AKR2A captures its clients at ribosomes during translation. This is similar to the behaviour of the ER-targeting factors SRP and pre-targeting complex Bat3/TRC35/Ubl4A, and the cytosolic chaperones that assist the folding of nascent proteins [36] , [45] , [46] , [47] , [48] , [49] . Together with previous work on SRP and pre-targeting complex Bat3/TRC35/Ubl4A, our study suggests that ribosomes serve as a platform for the docking of cytosolic factors that target organellar proteins. AKR2A has a basal binding affinity for ribosomes. This binding affinity is enhanced when ribosomes translate AKR2A clients. The data indicate that AKR2A binds ribosomes before the targeting signal of nascent AKR2A clients emerges from the ribosomal exit tunnel. One possible scenario is that AKR2A binds to ribosomes via the ARD at an early stage of translation, and subsequently captures its clients via the N-terminal domain at a later stage when they emerge from ribosomes but before they are released ( Fig. 8 ). This is an elegant mechanism for client protein sorting by factors involved in organellar protein targeting. This process is reminiscent of SRP action in ER targeting, in which SRP-binding affinity for ribosomes is greater when ribosomes are engaged in translation of SRP clients [50] . 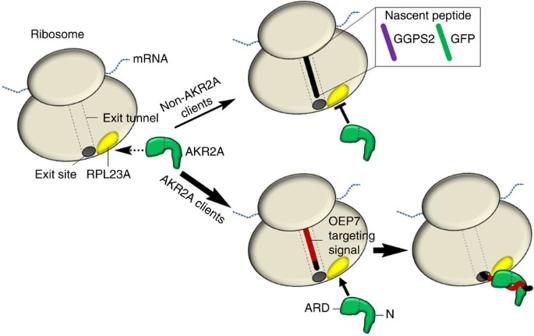Figure 8: Model for AKR2A binding to nascent AKR2A clients and RPL23A located at the ribosomal exit site. AKR2A has a basal binding affinity for ribosomes. The AKR2A ribosomal binding affinity is enhanced when the targeting signal of a nascent AKR2A client resides in the ribosomal exit tunnel before it emerges from the ribosome. In this process, AKR2A docks to RPL23A at the ribosomal tunnel exit site, and thereby is positioned for binding cargo proteins. After the targeting signal emerges from the exit tunnel, AKR2A simultaneously binds two RNC sites, ribosomal RPL23A and the COM client targeting signal. ARD=the C-terminal ankyrin repeat domain; N=the N-terminal AKR2A domain. Figure 8: Model for AKR2A binding to nascent AKR2A clients and RPL23A located at the ribosomal exit site. AKR2A has a basal binding affinity for ribosomes. The AKR2A ribosomal binding affinity is enhanced when the targeting signal of a nascent AKR2A client resides in the ribosomal exit tunnel before it emerges from the ribosome. In this process, AKR2A docks to RPL23A at the ribosomal tunnel exit site, and thereby is positioned for binding cargo proteins. After the targeting signal emerges from the exit tunnel, AKR2A simultaneously binds two RNC sites, ribosomal RPL23A and the COM client targeting signal. ARD=the C-terminal ankyrin repeat domain; N=the N-terminal AKR2A domain. Full size image The dynamics of AKR2A–ribosome interaction during translation raises an intriguing question of how nascent polypeptides residing in the exit tunnel can specifically induce ribosomal binding of their targeting factors. Recent work proposed that different nascent polypeptides may interact differently with the exit tunnel, which is lined primarily with negatively charged RNA molecules and ribosomal proteins RPL4, RPL17 and RPL39 [26] , [51] . The interaction between the nascent polypeptide and the exit tunnel may depend on individual amino acids and/or local structures of the nascent polypeptide residing in the exit tunnel. Consistent with this notion, different targeting signals have different amino acid compositions. The TMD of COM proteins has lower hydrophobicity than that of ER proteins [52] . Recent studies have suggested that the presence of a signal-anchor sequence within the exit tunnel of the ribosome promotes binding of SRP to the ribosome [50] . The dynamics of the SRP–ribosome interaction is affected by the biophysical properties of the nascent polypeptide located within the exit tunnel of the translating ribosome. Moreover, the presence of a transmembrane segment within the exit tunnel of the ribosome has been shown to promote recruitment of RAMP4 via RPL17 [53] . Thus, it appears that nascent chains within the exit tunnel of the ribosome are able to modulate the biochemical properties of the exit region of the tunnel and downstream events. In accordance with this idea, AKR2A was recruited to ribosomes only when the targeting signal of its client protein was passing through the interior of the exit tunnel of the ribosome during translation. We propose that, during the passage of targeting signals of nascent proteins through the exit tunnel, the different physicochemical properties of targeting signals may induce targeting signal-specific structural changes in the ribosome and/or in ribosomal proteins located at the exit site, thereby allowing the ribosome and/or certain ribosomal proteins to serve as a platform for interactions with targeting factors or chaperones of organellar protein targeting or protein folding, respectively. Multiple ribosomal proteins located at the exit region of the ribosomal tunnel have been shown to interact with various factors involved in organellar protein targeting or co-translational protein folding. RPL23 interacts with multiple factors such as SRP, chaperones and NAC, which raises the possibility that RPL23 functions as the general docking site. SRP and chaperones [35] , [54] also interact with RPL29 located at the exit region of the ribosomal tunnel. Zuotin, a component of the Hsp70- and Hsp40-based triad complex (Ssb/Ssz/Zuotin), which is involved in co-translational folding of nascent polypeptides in yeast, interacts with another ribosomal protein RPL31 (refs 55 , 56 ). AKR2A binds to RPL23A, the general docking site of multiple proteins. AKR2A and SRP may bind to two different sites on RPL23A in Arabidopsis . Similarly, Trigger factor and SRP simultaneously bind to two different sites on RPL23 [36] , [57] , [58] . The importance of RPL23A in protein targeting to chloroplasts was examined using Dex-inducible RPL23A -amiRNA plants. Consistent with the biochemical data, Dex-treated RPL23A -amiRNA plants exhibited yellow or albino phenotypes with severe defects in chloroplast protein targeting and chloroplast development. However, SRP-mediated protein targeting to the ER in Dex-treated RPL23A -amiRNA plants was essentially the same as that in control plants. In the case of SRP, the SRP54 N-domain binds to both RPL23 and RPL29 located at the exit region of the ribosomal tunnel [33] , [35] , [36] , [44] . Thus, although it is not fully understood how SRP can deliver proteins to the ER in Dex-treated RPL23A -amiRNA plants, one possible explanation is that in the absence of RPL23A, RPL29 alone may manage to recruit SRP to the ribosome for the SRP-mediated targeting of ER proteins in Dex-treated RPL23A -amiRNA plants. In addition to AKR2A binding to ribosomes, AKR2A binds to the nascent polypeptide as soon as the targeting signal emerges from the ribosomal exit tunnel. In fact, AKR2A binding to RPL23A at the ribosomal exit site induces AKR2A binding to its client when it emerges from the ribosome. The mode of interaction between AKR2A and RNCs may change depending on the stage of translation. AKR2A initially binds to ribosomes; subsequently, after the targeting signal emerges, it binds simultaneously to both ribosomes and clients. When translation is complete, AKR2A binds only to the client protein. The interaction between AKR2A and its clients during translation is crucial for protein targeting to chloroplasts in two different ways. First, it greatly improves the sorting efficiency of COM proteins among nascent proteins. Second, it eliminates the potential nonspecific aggregate formation of COM proteins in the aqueous cytosol before they are targeted to the chloroplast [8] , [59] . AKR2s are involved in the targeting of COM-localized signal-anchored (SA) proteins OEP7 and Toc64 as well as tail-anchored (TA) proteins Toc33/Toc34 and OEP9 [2] , [8] , [9] . In Dex-treated RPL23A -amiRNA plants, COM proteins Toc75 and Toc159 as well as stromal protein RbcS and thylakoid protein Lhcb4 were also reduced in their levels. It is possible that lower levels of Toc components involved in protein import result in reduced levels of transit peptide-containing proteins such as Toc75, RbcS and Lhcb4 in Dex-treated RPL23A-amiRNA plants. Thus, AKR2A-mediated protein targeting directly or indirectly plays a crucial role in chloroplast proteome biogenesis. Materials The silane coupling agent, N-[3-(triethoxysilyl)propyl]-O-polyethyleneoxide urethane (TPU) (Gelest), was stored under nitrogen, and all other chemicals and solvents were reagent grade from Sigma-Aldrich unless noted otherwise. All washing solvents for the probes and substrates were HPLC grade from Mallinckrodt Baker. Ultrapure deionized (DI) water (18.2 MΩ cm) was produced by the Milli-Q purification system (Millipore). The silicon-nitride probes (PEN-0012-03; k = ∼ 16 pN nm −1 ) were purchased from NanoInk. The polished prime Si(100) wafers (dopant, phosphorus; resistivity, 1.0–10.0 Ω cm) were purchased from Silicon Quest International. All water used in the ribosomal complex experiments was pretreated overnight with diethylpyrocarbonate [0.05% (v/v)]. Plant growth Arabidopsis plants (Col-0) were grown on Murashige-Skoog (MS) plates or liquid media supplemented with 1% sucrose in a growth chamber at 20–22 °C under a 16 h light/8 h dark cycle. Leaves or whole tissues were harvested from 10-day- to 3-week-old plants and used immediately for protoplast isolation or total RNA extraction. Construction of plasmid DNAs The constructs of GST- or His-tagged recombinant proteins RPL23A , RPL32A and OEP7 deletion mutants were generated using a PCR approach. The primer sequences used in this study are listed in Supplementary Table 5 . The primers used were as follows: RPL23aA-F1 and RPL23aA-R1 for His:RPL23aA ; RPL23aB-F1 and RPL23aB-R1 for His:RPL23aB ; RPL32A-F and RPL32A-R for His:RPL32A ; RPL23aA-F2 and RPL23aA-R2 for GST:RPL23aA ; RPL23aB-F2 and RPL23aB-R2 for GST:RPL23aB ; OEP7-F1 and OEP7(9)-R for GST:OEP7(9) ; OEP7-F1 and OEP7(27)-R for GST:OEP7(27) ; OEP7-F1 and OEP7(36)-R1 for GST:OEP7(36) ; and OEP7-F1 and OEP7(50)-R1 for GST:OEP7(50) . PCR products were ligated to pRSET-A for His tagging or pGEX5x1 for GST tagging. The primers used for generation of in vitro translation constructs were as follows: OEP7-F2 and OEP7(36)-R2 for OEP7(36) ; GFP-F1 and GFP(36)-R for GFP(36) ; GGPS2-F and GGPS2(36)-R for GGPS2(36) ; BiP-F and BiP-R for BiP(36) ; and AtToc64-F and AtToc64-R for AtToc64(36) . To generate OEP7:GFP(90) and OEP7:GFP(104) , PCR was performed using OEP7-F2/OEP7(50)-R2 and GFP-F2/GFP(40)-R for the first PCR of OEP7:GFP(90); OEP7-F2/OEP7-R2 and GFP-F3/GFP(40)-R for the first PCR of OEP7:GFP(104); and OEP7-F2 and GFP(40)-R for the second PCR of OEP7:GFP(90) and OEP7:GFP(104). The PCR products were ligated into the vector. To generate AtToc64:HA , PCR was performed using AtToc64-F2 and AtToc64-HA-R and 326-AtToc64:GFP as a template. The PCR product was ligated into pCS2+ for in vitro transcription. Construction of His:AKR2A , His:AKR2A(1−210) , His:ARD(211−342) , His:GFP , GST:AKR2A , GST:OEP7 , HA:AKR2A and AtOEP7:GFP was described previously [8] , [60] , [61] . The RPL23A -amiRNA construct was designed using Web MicroRNA Designer 3 ( http://wmd3.weigelworld.org ). The RPL23A -amiRNA was prepared by overlapping PCR as described previously [62] . The primer sets used were RPL23A-I miR-s, RPL23A-II miR-a, RPL23A-III miR*s and RPL23A-IV miR*a, together with two vector primers (amiRNA-A and amiRNA-B) in the adjacent region that defines the amiRNA foldback. The resulting PCR fragment, including the full amiRNA foldback, was ligated into the inducible vector pTA7002. The control-amiRNA vector was described previously [63] . All PCR products were sequenced to confirm the nucleotide sequences. Transient expression of proteins in protoplasts Plasmids were purified using the HiPure Plasmid DNA Purification kit (Invitrogen, Carlsbad, CA) according to the manufacturer’s protocol. The fusion constructs were transformed into protoplasts prepared from whole Arabidopsis seedlings using polyethylene glycol-mediated transformation [64] , [65] . Generation of transgenic Arabidopsis plants Transgenic plants were generated by the floral dipping method [66] . Transgenic plants were screened on MS medium containing 1% sucrose and antibiotics (30 mg l −1 hygromycin B and 100 mg l −1 cefotaxime), and homozygous lines were isolated at the T3 generation. RNA extraction and quantitative RT-PCR For quantitative RT-PCR, total RNA was isolated from 10-day-old seedlings grown in MS liquid medium supplemented with 1% sucrose in a growth chamber at 20−22 °C under a 16 h light/8 h dark cycle. Total RNA was extracted using the RNAqueous kit (Ambion, Austin, TX). TURBO DNase (Ambion, Austin, TX) was used to remove any DNA contamination from the RNA samples, and extracted RNA was used for reverse transcription into cDNA using the High Capacity cDNA Reverse Transcription kit (AB, Foster City, CA). Quantitative RT-PCR was performed with a SYBR green kit (AB) to detect RPL23aA , RPL23aB and ACT2 . Amplified samples were normalized with ACT2 . The primers used were RPL23aA-RT-F and RPL23aA-RT-R for RPL23aA , RPL23aB-RT-F and RPL23aB-RT-R for RPL23aB , and ACT2-F and ACT2-R for ACT2 . Preparation of RNCs and ribosome-binding assay We generated RNCs using the transcription and translation-coupled wheat-germ extract systems (Promega). For transcription by T7 polymerase, linearized DNA template containing a T7 promoter was prepared by PCR using the following T7 Pro(−200) and reverse primers: OEP7(36)-T for OEP7(36) ; GFP(36)-T for GFP(36) ; GGPS2(36)-T for GGPS2(36) ; BiP(36)-T for BiP(36) ; AtToc64(36)-T for AtToc64(36) ; and GFP(40)-T for OEP7:GFP(90) and OEP7:GFP(104) . PCR products were expressed according to the manufacturer’s protocol. For RNA labelling, 1 μM biotin-11-CTP (Roche) was added to the reaction mixture. For ribosome-binding assay, purified His:AKR2A (0.25 μM) was added to the reaction mixture and incubated for 60 min at 30 °C. RNCs or His:AKR2A-bound RNCs were separated from the rest of the wheat-germ extract by ultracentrifugation through a 20% sucrose cushion using a TLA 120.2 rotor for 90 min at 200,000 × g . The recovered samples were subjected to AFM analysis or western blot analysis. To label nascent polypeptides, we used EasyTag Express Protein Labelling Mix supplemented with [ 35 S]methionine and [ 35 S]cysteine (Perkin Elmer). EasyTag Express Protein Labelling Mix (4 μl) was added to the reaction mixture. After incubation, free radio-labelled amino acids were removed using PD-10 desalting columns. The samples were separated by 18% SDS–PAGE after boiling in sample loading buffer. After electrophoresis, the gels were dried and subjected to autoradiography. Recombinant protein purification and protein pull-down assay E. coli BL21 (DE3) cells transformed with different constructs encoding GST- or His-fused recombinant proteins were cultured to OD 600 ≈0.6. Protein expression was induced by adding 0.5−1 mM IPTG at 37 °C for 3 h. GST or GST-fusion proteins were bound to glutathione beads (Thermo Scientific, Rockford, IL) and washed several times with buffer (50 mM Tris-HCl, pH 7.5, 150 mM NaCl, 5 mM EDTA, 1% Triton X-100, 1 × complete protease inhibitor cocktail (Roche, Werk Penzberg, Germany)) for purification. His-tagged proteins were bound to Ni + -NTA agarose beads (Qiagen, Hilden, Germany) and washed several times with washing buffer (50 mM NaH 2 PO 4 , pH 8.0, 300 mM NaCl, 10 mM imidazole, 1% Triton X-100, 1 × complete protease inhibitor cocktail (Roche)) for purification. To study the interaction of RPL23A with AKR2A, in vitro protein pull-down experiments were performed. In brief, GST alone or GST:AKR2A (3 μg) immobilized on glutathione beads was incubated with His-tagged recombinant proteins (1 μg) as prey in binding buffer (20 mM Tris-HCl, pH 7.5, 150 mM NaCl, 3 mM MgCl 2 , 1 mM DTT, 0.1% Triton X-100) at 4 °C for 3 h. Beads were washed three times with binding buffer. Subsequently, proteins were separated by SDS–PAGE and analysed by western blotting using an anti-His antibody (dilution 1:1,000, Qiagen, Cat. No. 34610). Polysome analysis The AtToc64:HA DNA fragment was amplified by PCR using 5′-pCS2-transcription (5′-CGCCATTCTGCCTGGGGAC-3′) and 3′-pCS2-transcription (5′-CAATAGCATCACAAATTTCACAAA-3′) as the primer set and pCS2+AtToc64:HA plasmid as a template. Capped and polyadenylated AtToc64:HA mRNAs were generated by mMESSAGE mMACHINE SP6 (Ambion) according to the manufacturer’s protocol. AtToc64:HA mRNA (2 μg) and purified His:AKR2A (0.25 μM) were added to the wheat-germ extract system (Promega) and incubated for 60 to 90 min at 30 °C. After incubation, cycloheximide (0.1 mg ml −1 ) was added to terminate translation. A 15−50% (w/v) linear sucrose gradient was prepared using the method of Abe and Davies [67] . In vitro translation mixtures (0.2 ml) were loaded onto the top of the linear sucrose gradients, and ribosomes were fractionated by ultracentrifugation at 200,000 × g for 120 min at 4 °C in a SW 41 Ti rotor (Beckman). The gradient was collected from the top to the bottom with a density gradient fractionator RETRIEVER 500 (Teledyne Isco) in a total of 20 fractions (each fraction with 500 μl), and these fractions were analysed by measuring absorbance at 254 nm. Data were recorded and processed with UA-6 (Teledyne Isco). Subsequently, these fractions were subjected to TCA precipitation, the pellets were re-suspended in 0.1 N NaOH, and then analysed by western blotting using anti-RPL23A (dilution 1:1,000, Abcam, Cat. No. ab71341) and anti-His antibodies. Co-immunoprecipitation and crosslinking For co-immunoprecipitation analyses, in vitro translation samples were incubated with 2 μg of an anti-His monoclonal antibody (Qiagen) for 2 h at 4 °C, followed by an additional incubation with 20 μl of protein-A Sepharose CL-4B beads (Amersham Biosciences) for 2 h at 4 °C. Immunoprecipitates were washed three times with immunoprecipitation buffer (50 mM HEPES, pH 7.5, 150 mM NaCl, 3 mM MgCl 2 , 1 mM DTT, 0.5% Triton X-100) and subjected to RNA isolation. His:AKR2A-bound RNCs were treated with crosslinker BS(PEG) 9 (Pierce Biotechnology, Rockford, IL, USA) according to the manufacturer’s instructions. Western blot analysis was performed with specific antibodies [68] . Immunoblotting analysis Proteins were separated by 8 ∼ 12% SDS–PAGE after boiling in the sample loading buffer, and the gel was transferred onto a polyvinylidene fluoride membrane (Millipore Corporation, USA). For western blot analysis, the membranes were treated with 6% non-fat dry milk in TTBS buffer for 30 min to prevent nonspecific binding of antibodies followed by incubation with corresponding primary and secondary antibodies using standard protocols. The antibodies used in this study include anti-AALP (dilution 1:3,000), anti-actin (dilution 1:1,000, MP Biomedicals, Cat. No. 69100), anti-AKR2 (dilution 1:1,000), anti-BiP (dilution 1:3,000), anti-catalase (dilution 1:1,000), anti-GFP (dilution 1:1,000, Clontech, Cat. No. 632381), anti-HA (dilution 1:1,000, Roche, Cat. No. 11 867 423 001), anti-Hsp70 (dilution 1:3,000, Agrisera, Cat. No. AS08 371), anti-Lhcb4 (dilution 1:7,000, Agrisera, Cat. No. AS04 045), anti-PIP2 (dilution 1:1,000, antibodies-online GmbH, Cat. No. ABIN349672), anti-RbcS (dilution 1:5,000, Agrisera, Cat. No. AS07 259), anti-RPL32 (dilution 1:1,000, Abcam, Cat. No. ab50759), anti-SRP54 (dilution 1:1,000, BD Biosciences, Cat. No. 610940), anti-Toc34 (dilution 1:5,000, Agrisera, Cat. No. AS07 238), anti-Toc75 (dilution 1:5,000, Agrisera, Cat. No. AS06 150), anti-Toc159 (dilution 1:5,000, gift from Dr Hsou-min Li, Academia Sinica, Taiwan), anti-VDAC1 (dilution 1:5,000, Agrisera, Cat. No. AS07 212), anti-VSR (dilution 1:1,000), anti-mouse horseradish peroxidase-conjugated antibody (dilution 1:7,000, Bethyl, Cat. No. A90-146P), anti-rabbit horseradish peroxidase-conjugated antibody (dilution 1:7,000, Bethyl, Cat. No. A120-101P) and anti-rat horseradish peroxidase-conjugated antibody (dilution 1:7,000, Bethyl, Cat. No. A110-105P). Full-size images are presented in Supplementary Figs 13 and 14 . Immobilization of proteins on AFM probes and substrates Dendron-modified AFM probes and substrates were prepared and conjugated with reduced glutathione (GSH) [29] . GSH-tethered probes were immersed in PBS buffer (10 mM phosphate buffer, 2.7 mM KCl, 137 mM NaCl, 3 mM MgCl 2 , pH 7.4) to solubilize GST-fused AKR2A (32 μg ml −1 ); probes were immersed for 30 min at room temperature. For preparation of the reference systems, GSH-tethered substrates were placed in PBS buffer to solubilize GST-fused OEP7 deletion mutants ( ∼ 15.5 μg ml −1 ), or GST-fused RPL23aA and RPL23aB ( ∼ 22.2 μg ml −1 ); substrates were immersed for 30 min at room temperature. After incubation, the probes and substrates were rinsed with the same buffer and stored in the buffer. RNC immobilization on dendron-modified substrates Dendron-modified substrates were placed in 50 mM NaHCO 3 buffer (pH 8.5) with a small amount of dimethylformamide (DMF) to solubilize biotinyl-N-hydroxy-succinimide (NHS-biotin) (10 mM) and incubated for 2 h. Then, substrates were immersed in DMF and the solution was stirred for 30 min at room temperature. Subsequently, substrates were rinsed thoroughly with DMF, then with methanol and then dried under vacuum. The resulting substrates were placed in PBS buffer (10 mM phosphate buffer, 2.7 mM KCl, 137 mM NaCl, pH 7.4) to solubilize streptavidin (30 μg ml −1 ) for 30 min at room temperature. After incubation, substrates were washed briefly with PBS buffer (10 mM phosphate buffer, 2.7 mM KCl, 137 mM NaCl, 3 mM MgCl 2 , 0.05% (v/v) DEPC, pH 7.4) and placed in PBS buffer to solubilize RNCs at room temperature for 30 min. RNCs were diluted with a 40 × volume of PBS buffer. Finally, substrates were rinsed with the same buffer and stored in the buffer. Recording force-distance curves NanoWizard I AFM (JPK Instrument AG) was used for force measurement of the reference systems and the RNC samples. ForceRobot 300 automated force spectroscope (JPK Instrument AG) was employed for force mapping the RNC samples. In both cases, the force-distance curves were recorded at a retraction speed of 540 nm s −1 . All curves were measured at room temperature in PBS buffer containing 3.0 mM MgCl 2 (for the reference systems) or 3.0 mM MgCl 2 and DEPC (0.05% (v/v)) for ribosome samples. The spring constant of each AFM probe was calibrated in solution using JPK SPM software (thermal-noise method), and the resulting value ranged from 15 to 25 pN nm −1 . For each sample, at least three independent measurements were conducted using freshly prepared probe and substrate for each measurement. To obtain the most probable force value for the unbinding event, more than 100 force-distance curves were recorded at a position, and more than three positions on a substrate were examined in each experiment. The collected force-distance curves were analysed using the JPK data processing software. An unbinding force histogram was generated from the whole set of the collected specific curves. For the double-peaked curves, the force value of the larger peak was used to generate the force histogram. The most probable force value was obtained by fitting with a single Gaussian curve, and the presented statistical error was 2 σ /√ N , where 2 σ was the width of the distribution and N was the number of unbinding events in the histogram [18] . Force mapping and data analysis for RNCs Adhesion force maps were obtained by processing the force value recorded during raster-scanning on a 300 nm × 300 nm area with a pixel size of 15 nm. The force-distance curves were recorded five times at each pixel, and the force value from the specific curves was averaged. To generate a map, a pixel that did not show any specific curve or that showed a specific curve only once out of five measurements was not included. Dynamic force spectroscopy for reference systems A z -scan length of 450 nm and z -scan rates of 0.023−10.0 Hz were used, resulting in loading rates of 200 to 200,000 pN s −1 . The loading rate was determined by multiplying the retraction speed by the effective spring constant. The kinetic off rate constant ( k off ) and the energy barrier distance ( x β ) were obtained from the equation, F* = f β ln( r / k off f β ), where f β is the ratio of the thermal energy k B T to the length scale x β [69] . Electron microscopy Arabidopsis leaf tissues were fixed with 2% paraformaldehyde and 2% glutaraldehyde in 50 mM cacodylate buffer (pH 7.2) for 4 h, washed with the same buffer and post-fixed with 1% osmium tetroxide in cacodylate buffer for 2 h. After dehydration, leaf specimens were embedded in LR White (London Resin). Ultrathin sections of leaf specimens (60−80 nm thick) were collected on uncoated copper grids (150 mesh), and then stained with 3% uranyl acetate and Reynolds’ lead citrate. Images were captured with a transmission electron microscope (Jeol JEM-1011) at 80 kV. Statistical analysis Data are expressed as a mean value±s.d. or s.e.m. No statistical method was used to predetermine sample sizes. Statistical significance was examined using the Student’s two-tail t -test. A P value <0.05 was considered statistically significant. In figures with quantitative data, * designates P <0.05, ** P <0.01, and *** P <0.001. How to cite this article: Kim, D. H. et al. Cytosolic targeting factor AKR2A captures chloroplast outer membrane-localized client proteins at the ribosome during translation. Nat. Commun. 6:6843 doi: 10.1038/ncomms7843 (2015).